Mesoporous silicon sponge as an anti-pulverization structure for high-performance lithium-ion battery anodes Nanostructured silicon is a promising anode material for high-performance lithium-ion batteries, yet scalable synthesis of such materials, and retaining good cycling stability in high loading electrode remain significant challenges. Here we combine in-situ transmission electron microscopy and continuum media mechanical calculations to demonstrate that large (>20 μm) mesoporous silicon sponge prepared by the anodization method can limit the particle volume expansion at full lithiation to ~30% and prevent pulverization in bulk silicon particles. The mesoporous silicon sponge can deliver a capacity of up to ~750 mAh g −1 based on the total electrode weight with >80% capacity retention over 1,000 cycles. The first cycle irreversible capacity loss of pre-lithiated electrode is <5%. Bulk electrodes with an area-specific-capacity of ~1.5 mAh cm −2 and ~92% capacity retention over 300 cycles are also demonstrated. The insight obtained from this work also provides guidance for the design of other materials that may experience large volume variation during operations. Increasing demands for high energy density, long cycle life, and low-cost lithium (Li)-ion batteries in critical applications such as electrical vehicles and portable devices have stimulated extensive research interest in developing novel electrode materials [1] , [2] . Among all the candidates for anode materials, silicon (Si) has a theoretical specific capacity of ~4,200 mAh g −1 (Li 22 Si 5 ), ~11 times of the theoretical specific capacity of the state-of-the-art graphite anode, and it does not have the safety concern of lithium metal dendrite formation [3] . Therefore, Si has been regarded as one of the most promising anode materials for next-generation Li-ion batteries. However, its large volume expansion (>300%) during the lithiation process leads to the pulverization of silicon particles (>200 nm) and subsequently results in fast capacity fade of the electrode [3] . Many in-situ studies have directly observed the intrinsic volume expansion and pulverization of Si particles [4] , [5] , [6] . To overcome/bypass the pulverization problem, tremendous effort has been made on the synthesis of ultra-fine Si nanoparticles (<50 nm), development of new binders, and design of novel nanostructured Si materials, such as nanowires, nanotubes, hollow spheres and core-shell structures [7] , [8] , [9] , [10] , [11] , [12] , [13] , [14] , [15] , [16] , [17] , [18] , [19] , [20] , [21] , [22] , [23] , [24] , [25] , [26] , [27] , [28] , [29] , [30] , [31] , [32] . Milestone performance with a capacity of ~600 mAh g −1 and ~88% capacity retention over 6,000 cycles at a 12C rate has been demonstrated with double-walled Si nanotubes at a low mass loading [11] . Recently, over 100 stable cycles has also been demonstrated with a high loading Si anodes using pomegranate-like Si-C yolk-shell structures [33] . However, scalable synthesis of nanostructured Si materials that retain good long-term cycling stability in bulk electrodes of high mass loading remains a significant challenge. In general, the cycling stability of nanostructured Si anodes degrades rapidly as the mass loading or the electrode thickness increases to >10 μm. Methods are needed to prepare bulk Si materials without structural degradation during lithiation/de-lithiation. Recently, porous structured Si and Si-based composites have attracted significant attention [14] , [24] , [25] , [26] , [27] , [28] , [29] , [30] , [31] , [32] . The idea is to pre-form meso/macropores in the Si structure to accommodate the large volume expansion that accompanies the lithiation process. Newly developed synthetic chemistries and approaches that lead to significantly improved performance have been demonstrated. However, the suppression of pulverization of bulk Si particles, and long-term cycling stability at high Si loading conditions have not been demonstrated. The existing work on Si anodes has not yet met the requirements for commercial applications because of unsatisfactory performance or serious challenges associated with cost and scale-up. In this study, we synthesize large (>20 μm) mesoporous Si sponge (MSS) using an electrochemical etching method and demonstrated its excellent performance as anodes for Li-ion batteries. The MSS has a highly porous structure with thin crystalline Si walls surrounding large pores that are up to ~50 nm in diameter. In-situ transmission electron microscopy (TEM) shows that the volume change of the Si walls during the charge/discharge processes is primarily accommodated by the inner pores in the MSS, leading to only ~30% expansion in the full particle size instead of >300% expansion as in the case of conventional Si particles, and the particles do not pulverize even after one thousand charge/discharge cycles. With this unique structure, a MSS anode delivers a capacity of up to ~750 mAh g −1 based on the whole electrode weight including binder and conductive carbon, and retains more than 80% capacity over 1,000 cycles. Its first cycle irreversible capacity loss can be reduced to <5% by pre-lithiation with Li powder. The MSS-based anode also demonstrates ~92% capacity retention over 300 cycles at a high area-specific-capacity of ~1.5 mAh cm −2 . Furthermore, the thick electrodes with an areal capacity of ~3 and 4 mAh cm −2 also demonstrate a capacity retention of >96% over 70 cycles. These results suggest that stable bulk Si anode materials are possible even at deep lithiation and high loading conditions required for practical applications. Calculation of the MSS volume expansion The large volume expansion of Si during lithiation is intrinsic; however, the effects of the expansion such as the pulverization of bulk/micron-sized Si particles can be alleviated or eliminated by rational design of the Si structure. With the help of theoretical calculations, we identified a MSS structure with inner pores that can accommodate most of the volume change so that the overall particle experiences minimal expansion. 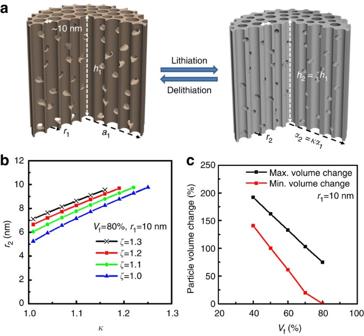Figure 1: The MSS model structure and theoretical estimation of its structure change after lithiation. (a) A schematic model of the MSS particle. (b) The correlation of the pore radius after full lithiation (r2), and the expansion rates of the particle along the radical direction (κ) and along the axial direction (ξ).r1=10 nm;Vf=80%. The silicon wall thickness is 10 nm. (c) The plot of the MSS particle volume expansion versus porosity (Vf).r1=10 nm. The Si wall thickness is 10 nm. Figure 1a schematically illustrates the structural change of a model of cylindrical MSS particle with cylindrical pores during the lithiation/de-lithiation processes. The solid Si portion of the particle is predicted to experience a ~300% volume increase at the full lithiation state. However, the dimension ( a , h ) of the particle experiences only a small increase/expansion during lithiation if the void/pore radius ( r ) decreases sufficiently. Based on the assumption of stress-free or volume conservation, the effect of the initial pore radius ( r 1 ) and the porosity/void volume fraction ( V f ) on the average volume change can be estimated and optimized. For a MSS particle ( a 1 , h 1 ) with given porosity ( V f =80%), Si wall thickness (~10 nm), initial pore radius ( r 1 =10 nm), the expansion rates of the cylindrical particle along the radial direction ( κ ), along the axial direction ( ξ ) and the pore radius after lithiation ( r 2 ) are calculated and plotted in Fig. 1b . The pore volume after full lithiation is predicted to be 75% less and the radius ( r 2 ) will be approximately half of the initial pore radius assuming the overall particle does not expand at all (in real cases, the ratio of the expansion towards the inner pores and outside dimensions depends on the Li-ion diffusion and other factors such as the structure confinement effect). Similarly, we estimated the upper and lower bounds of particle volume changes as a function of V f and initial pore radius ( r 1 ) under the following constraint conditions: r 2 ≥0, κ ≥1 and ξ ≥1. Figure 1c shows that the overall volume expansion decreases almost linearly with the increase of void volume fraction ( V f ) in the MSS particle. The volume change decreases to between 0 and 75% if the MSS particle has ~80% porosity ( V f =80%), thin Si walls of ~10 nm and large initial pore radius ( r 1 =10 nm). Systematic calculations on the influence of porosity ( V f ) and initial pore radius ( r 1 ) on the particle volume expansion were performed; the results are given in the Supplementary Figs 1 and 2 . Figure 1: The MSS model structure and theoretical estimation of its structure change after lithiation. ( a ) A schematic model of the MSS particle. ( b ) The correlation of the pore radius after full lithiation ( r 2 ), and the expansion rates of the particle along the radical direction ( κ ) and along the axial direction ( ξ ). r 1 =10 nm; V f =80%. The silicon wall thickness is 10 nm. ( c ) The plot of the MSS particle volume expansion versus porosity ( V f ). r 1 =10 nm. The Si wall thickness is 10 nm. Full size image Preparation and characterization of the desired MSS structure The preparation of porous Si by anodic electrochemical etching of crystalline Si has been known for more than 50 years [34] . The process allows the designed fabrication of various pore sizes (between 2 nm to several μm) and porosities (ranging from 5–95%) and it has been exploited for applications such as bio-imaging reagents and controlled drug delivery [35] , [36] , [37] . Here we tailored the etching protocol to synthesize MSS with a high porosity suitable for rechargeable Li-ion battery applications (See Methods). 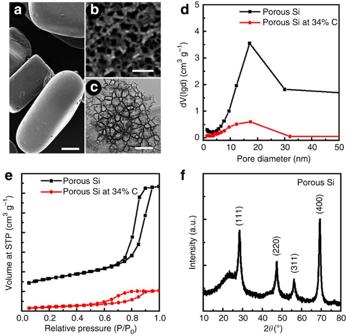Figure 2: Structure of the MSS. (aandb) SEM images of the MSS at different magnifications. (c) TEM image of the MSS. The scale bar ina,bandcis 20 μm, 100 nm and 100 nm, respectively. (d) and (e) Pore size distribution and isothermal curves of the MSS sample before and after carbon deposition. (f) XRD pattern of the MSS material. Figure 2a,b shows typical scanning electron microscope (SEM) images of the MSS. At low magnification ( Fig. 2a ), the MSS particles have the appearance of irregular bricks or rocks with overall dimensions of >~20 μm. The highly porous sponge-like structure of the particles is revealed at higher magnifications ( Fig. 2b ), in which large pores with diameters up to ~50 nm are surrounded by thin (~10 nm) Si walls. Figure 2c shows the TEM image of a thin slide from a bulk MSS particle. The pores are up to 50 nm in diameter surrounding with thin walls of ~8 nm, in consistent with the SEM results. High-solution TEM images ( Supplementary Fig. 3 ) show that the MSS wall consists of a crystalline Si skeleton coated with a thin amorphous silicon layer of ~1–3 nm in thickness. The thin amorphous layer is silicon oxide formed during exposure of the material to air. The energy-dispersive x-ray spectroscopy analysis shows that the MSS has ~19 wt% oxygen content (see Supplementary Method 1 ). This oxide layer may lower the capacity and induce first cycle irreversible capacity loss ( vide infra ). Figure 2: Structure of the MSS. ( a and b ) SEM images of the MSS at different magnifications. ( c ) TEM image of the MSS. The scale bar in a , b and c is 20 μm, 100 nm and 100 nm, respectively. ( d ) and ( e ) Pore size distribution and isothermal curves of the MSS sample before and after carbon deposition. ( f ) XRD pattern of the MSS material. Full size image Nitrogen gas sorption measurements ( Fig. 2d,e ) were conducted to investigate the pore size distribution, surface area and porosity of the MSS. The pore diameter of the MSS is ~17.1 nm ( Fig. 2d , calculated from the adsorption branch using the Barrett–Joyner–Halenda method; see detailed results in Supplementary Table 1 .) and the surface area is ~494.7 m 2 g −1 (calculated using the Brunauer–Emmett–Teller theory). The pore volume is ~1.7 cm 3 g −1 ( Supplementary Table 1 ) and hence the porosity is ~80%. This MSS closely approximates the calculated optimal structure. The x-ray diffraction (XRD) pattern ( Fig. 2f ) shows that the MSS consists of crystalline Si and amorphous oxide, in consistent with the TEM results ( Fig. 2c and Supplementary Fig. 3 ). To improve the electrical conductivity, the as-prepared MSS material was coated with amorphous carbon using chemical vapour deposition (see Methods) [38] . The Brunauer–Emmett–Teller surface area (155.8 m 2 g −1 ) and pore volume (0.33 cm 3 g −1 ) of the MSS significantly decreases ( Fig. 2d,e and Supplementary Table 1 ) after carbon coating, indicating that the carbon is deposited both inside the pores and on the surface of the MSS particles. Thermogravimetric analysis revealed a carbon content of ~34 wt% ( Supplementary Fig. 4 ). We believe that the carbon coating not only improves the conductivity of the MSS, but also mechanically/electrically integrates the particle during cycling. In-situ TEM experiment The volume expansion of the MSS particle under cycling conditions was quantitated by in-situ TEM during battery operation (see Methods). The in-situ TEM battery experiment is schematically shown in Fig. 3a . A carbon-coated MSS particle is loaded onto a Si nanowire, which is then connected to the Li 2 O/Li end. The Si nanowire lithiates first and transports Li to the MSS particle. As shown in Fig. 3b , the dimension of the pristine MSS particle is characterized by the length in two directions: parallel and perpendicular to the pore direction. The small red arrow in the Figure indicates the location on the particle where the measurement was performed. The dimension and crystallinity of MSS at different stages of lithiation were monitored by TEM ( Fig. 3b–e ). Before lithiation, the pristine particle was 1,219 nm in length (perpendicular to the pore direction) and 488 nm in width (parallel to the pore direction) ( Fig. 3b ). The corresponding selected area electron diffraction pattern indicates that the direction perpendicular to the pore direction is the <01-1> direction, which is consistent with the <100> orientation of pores typically observed with this type of porous Si [35] . As lithiation continued to 22 min ( Fig. 3c ), the length increased to 1295, nm while the width increased to 508 nm. The diffraction pattern at 22 min showed faint diffraction spots, indication of the lowering of crystallinity induced by the lithiation process. After 40 min of lithiation, the particle showed a completely amorphous structure as exhibited by the ring patterns of the diffraction pattern in Fig. 3d . At the same time, the length increased to 1,315 nm and the width increased to 530 nm. After an extended period of lithiation (160 min), the sample was fully lithiated. At this point the sample showed no further increase in length, and the width increased to 552 nm. The diffraction pattern at this final lithiation state indicated that the structure was amorphous, and the electron energy loss spectrum ( Supplementary Fig. 5 ) indicated a Li:Si atomic ratio of 3.75, which corresponds to full lithiation at room temperature [3] . 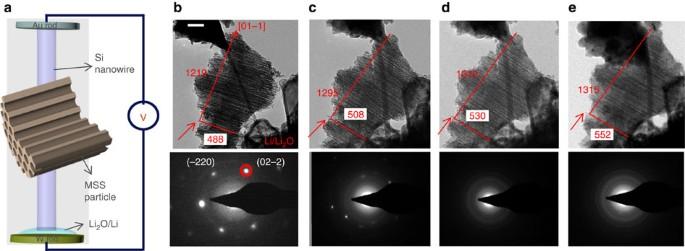Figure 3:In-situTEM observation of the lithiation process of an MSS particle. (a) Schematic figure of thein-situTEM battery experiment. (b–e) TEM images and selected area electron diffraction patterns of the MSS particle at different lithiation states: (b) before lithiation; (c) 22 min of lithiation; (d) 40 min of lithiation; (e) 160 min of lithiation. Scale bar, 200 nm (b–e). Figure 3: In-situ TEM observation of the lithiation process of an MSS particle. ( a ) Schematic figure of the in-situ TEM battery experiment. ( b – e ) TEM images and selected area electron diffraction patterns of the MSS particle at different lithiation states: ( b ) before lithiation; ( c ) 22 min of lithiation; ( d ) 40 min of lithiation; ( e ) 160 min of lithiation. Scale bar, 200 nm ( b – e ). Full size image Electrochemical performance To further corroborate the stability of the MSS structure against pulverization during lithium insertion/extraction processes, MSS particles have been used to prepare anode and tested in lithium batteries (see Methods). Unlike conventional micron-sized Si particles that exhibit fast capacity fading [3] , the micron-sized MSS demonstrated superior electrochemical performance. 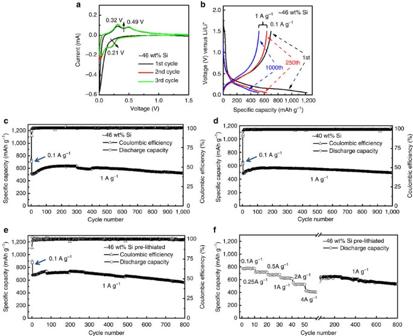Figure 4: Electrochemical performance of the MSS-based anodes. (a) Cyclic voltammogram curves of a typical MSS anode. (b) Typical charge–discharge profiles of the MSS anode with ~46 wt% MSS loading. (c) Long-term cycling of the MSS electrode inb. (d) Long-term cycling of an electrode with ~40 wt% MSS loading. (e) Long-term cycling of a pre-lithiated electrode with ~46 wt% MSS loading. (f) Rate performance of a pre-lithiated electrode with ~46 wt% MSS loading. Figure 4a shows the cyclic voltammetry curve of an anode prepared from the MSS material. The curves appear very similar to those obtained from standard crystalline Si [3] , [16] , and they are consistent with the crystalline XRD pattern shown in Fig. 2d . The cathodic peak at ~0.21 V and the anodic peaks at ~0.32 and ~0.49 V are characteristic of amorphous Si, and the cathodic peak at ~0 V is characteristic of both crystalline and amorphous Si [16] . In the first cathodic scan, only crystalline Si exists, so only one peak at ~0 V is observed. However, the crystalline structure becomes amorphous during lithiation, and hence, two anodic peaks of amorphous Si (at ~0.32 and ~0.49 V) are observed in the subsequent anodic scans. Figure 4: Electrochemical performance of the MSS-based anodes. ( a ) Cyclic voltammogram curves of a typical MSS anode. ( b ) Typical charge–discharge profiles of the MSS anode with ~46 wt% MSS loading. ( c ) Long-term cycling of the MSS electrode in b . ( d ) Long-term cycling of an electrode with ~40 wt% MSS loading. ( e ) Long-term cycling of a pre-lithiated electrode with ~46 wt% MSS loading. ( f ) Rate performance of a pre-lithiated electrode with ~46 wt% MSS loading. Full size image The charge-discharge curves ( Fig. 4b ) obtained between 0.05 and 1.5 V are similar to those observed with other nano-Si materials. A low Coulombic efficiency and relatively large irreversible capacity loss occurred during the first cycle, which is related to formation of the solid–electrolyte interphase and the high surface oxygen content in the surface of MSS and consistent with the amorphous signal appearing at 2θ=24° in the XRD pattern ( Fig. 2f ). The Coulombic efficiency for the electrodes without pre-lithiation treatment is ~56% in the 1st cycle and then it quickly increased to ~99.7%. The carbon-coated MSS displayed very good long-term cycling stability and a high capacity (up to ~750 mAh g −1 ). The specific capacity values reported in this work are based on the weight of the full electrode, including the MSS material, binder and carbon additive (see Methods). Figure 4c shows the representative results of an electrode with ~46 wt% MSS. It has a specific capacity of ~640 mAh g −1 and ~81% capacity retention over 1,000 cycles. By tuning the weight ratio of the MSS in electrodes, we can fine tune the capacity and the retention for different applications. Figure 4d shows the long-term cycling data for a battery with ~40 wt% MSS in the electrode. A capacity of ~570 mAh g −1 and ~87% capacity retention over 1,000 cycles were obtained ( Fig. 4d ). The capacity ramping-up process in the first 100 cycles can be attributed to the fact that the MSS has a large particle size; hence, it takes many cycles to fully utilize its full capacity. The large first cycle irreversible capacity loss, which would be a deficiency for practical applications, can be solved by pre-lithiation of the MSS anode (See detail pre-lithiation procedure and charge/discharge profile of pre-lithiated MSS in Supplementary Fig. 6 in the Supplementary Materials ). By adding an appropriate amount of stabilized Li metal powder (SLMP, FMC Lithium) to the MSS electrodes, the irreversible capacity loss in the first cycle was greatly reduced. As shown in Fig. 4e,f , pre-lithiated MSS electrodes displayed first cycle capacity losses as low as ~5% ( Fig. 4e ) and ~1% ( Fig. 4f ). The Coulombic efficiency for the electrodes with pre-lithiation treatment is ~94.5% for the 1st cycle and then it increased to >99.4%. As indicated in Fig. 4e,f , high capacities of ~740 mAh g −1 and ~650 mAh g −1 and ~80% capacity retention over 800 cycles were obtained. In spite of its large particle size, MSS particles have demonstrated very good rate performance. Figure 4f shows that the capacity is ~790 mAh g −1 at 0.1 A g −1 current density, ~630 mAh g −1 at 1 A g −1 , ~530 mAh g −1 at 2 A g −1 , and ~410 mAh g −1 at 4 A g −1 . The capacity retention is ~82% after 800 cycles (10 cycles each at current densities of 0.1, 0.25, 0.5, 1, 2, and 4 A g −1 and then 740 cycles at 1 A g −1 ), which demonstrates the ability of the MSS to recover after being subjected to high charge/discharge rates. Post-analysis of the electrode by SEM confirms the excellent structural stability of the MSS. As shown in Supplementary Fig. 7 , MSS particles before and after 1,000 cycles exhibit similar size (>20 μm) ( Supplementary Fig. 7a,b ) and size distribution ( Supplementary Fig. 7c ). The particles are coated with a layer of the solid–electrolyte interphase but they are not broken ( Supplementary Fig. 7b ). To further examine if cracks exist inside the large particles, we checked the cross-section of randomly picked large MSS particles after cycling. Supplementary Fig. 8 shows that the MSS particle still has similar porous structure and there is no cracking in the MSS after 1,000 cycles. With the pulverization eliminated and particle volume expansion limited to ~30%, the MSS material allows good cycling stability for electrodes with high Si loading per unit area. A high area-specific-capacity of ~1.50 mAh cm −2 at 0.5 mA cm −2 discharge and 0.75 mA cm −2 charge current density has been demonstrated ( Fig. 5a ). It shows excellent cycling stability with ~92% capacity retention over 300 cycles. The corresponding specific capacity is ~750 and 950 mAh g −1 at low current density of 0.06 mA cm −2 ( Supplementary Fig. 9 ). The pre-lithiated high loading MSS electrodes have very similar initial capacity while the cycling stability may be slightly different as a result of the hand-pressing pre-lithiation treatment procedure. Supplementary Fig. 10 shows another pre-lithiated electrode with an areal capacity of ~1.44 mAh cm −2 and ~90.7% capacity retention over 300 cycles. These thick electrodes without ( Supplementary Fig. 10a ) and with pre-lithiation treatment ( Supplementary Fig. 10b ) can have excellent extended cycling performance with ~85% capacity retention over 450 cycles. 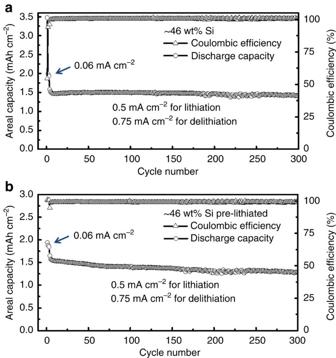Figure 5: Cycling stability of the MSS-based anodes with high areal discharge capacity of ~1.5 mAh cm−2. (a) A typical MSS anode. (b) A pre-lithiated MSS anode. Figure 5: Cycling stability of the MSS-based anodes with high areal discharge capacity of ~1.5 mAh cm −2 . ( a ) A typical MSS anode. ( b ) A pre-lithiated MSS anode. Full size image High loading electrodes with the areal capacity up to ~3 and 4 mAh cm −2 were also demonstrated. Supplementary Figure 11a shows the cycling performance of three cells with loading of ~3.5–4 mg cm −2 . The areal capacity is ~4.0 mAh cm −2 (3.7, 3.9 and 4.2 mAh cm −2 , respectively) at a charge/discharge current density of 0.06 mAh cm −2 and ~3 mAh cm −2 (2.6, 2.8 and 3.1 mAh cm −2 , respectively) at 0.5 mA cm −2 discharge and 0.75 mA cm −2 charge current density. The capacity retention is >96% after 70 cycles. With the loading further increased to ~5.3 mg cm −2 , the areal capacity can be >4 mAh cm −2 at 0.5 mA cm −2 discharge and 0.75 mA cm −2 charge current density ( Supplementary Fig. 11b ). We postulate that the suppression of pulverization and the low volume expansion of MSS particles are the result of three factors: (1) the pores in the MSS particle serve as buffers that accommodate the volume expansion of Si during lithiation; (2) the ~10 nm Si walls are sufficiently thin that they reversibly expand/shrink during lithiation/de-lithiation without breaking [7] ; and (3) the solid surface oxide layer formed at the pore wall surface serves to confine and reinforce the nanostructure [11] . We believe that these three factors together result in the unique structure of the MSS that leads to its desirable properties. This reasoning also explains the observation that the volume change revealed by the in-situ TEM study is somewhat smaller than those predicted by the theoretical calculations which does not count the effect of solid surface oxide layer. The calculations indicate that an optimal MSS particle should have a high porosity ( V f >70%), thin Si walls (thickness<~10 nm) and large pore radius ( r 1 >~10 nm) to preserve a relatively small overall volume variation (<75%) during lithiation/de-lithiation processes. It must be noted that the maximum volume expansion of the MSS particle only decreases 17% (from 75 to 58%) when the pore radius increases 150% from 10 to 25 nm. This suggests that ~10 nm pore radius can effectively accommodate the volume expansion. Further increase in pore size could lead to a decrease in the volumetric capacity of the electrode. It is well-known that Si shows significant anisotropic expansion upon lithiation, with an elongation of ~200% along the family of <011> directions [39] , [40] . Si particles with sizes >200 nm will pulverize during the lithiation process [4] , [5] . In the case of MSS, the channel of the pores in the porous Si is along <100> direction. Therefore, the expected large expansion of Si is along pore radius direction and can be absorbed by the open pores. This will effectively minimize the effect of volume expansion caused by lithiation process. In fact, the observed expansion for the whole particle along the <011> direction perpendicular to the pore channels is only ~7.8%. The small expansion observed along the pore direction (that is, <100> direction) is also consistent with the previous reports [39] , [40] . As a result, the MSS studied in this work exhibits the preferred pore orientation and pore structure which can effectively absorb the volume expansion inside of its nanostructure and prevent the particle from pulverization. For purpose of discussion we describe the three-dimensional MSS particle in terms of x , y , and z directions, where the x direction (<100>) is parallel to the pore direction and the y (<01-1>) and the z (<011>) directions are both perpendicular to the pore direction ( y and z are in the same direction family and have identical volume expansion.). The total volume expansion of the particle can be approximately written as x f * y f * z f − x 0 * y 0 * z 0 (where x f , y f , z f are the coordinates after full lithiation, while x 0 , y 0 , z 0 are the coordinates of the pristine state). The expansion along x , the pore direction (<100>), is 13.1%=(552−488)/488. The expansion along both y (<01-1>) and z (<011>) directions is 7.8%=(1315−1219)/1219. The apparent volume expansion of the particle is, therefore, calculated to be=( x f * y f * z f − x 0 * y 0 * z 0 )/( x 0 * y 0 * z 0 )=(1+13.1%)*(1+7.8%)*(1+7.8%)=~31.6%. It is much lower than the 300% volume increase of conventional dense Si particles. From these in-situ TEM observations, we conclude that the nanostructure of the MSS significantly reduces the apparent volume expansion and thus prevents lithiation-induced pulverization. The in-situ TEM results and the excellent electrochemical performance demonstrated above indicate that MSS has a great potential to be used as a high capacity, highly stable anode material in the next-generation Li-ion batteries. This study identified the desired microstructures for stable porous Si anodes. In addition to electrochemical etched single crystalline Si waver, porous Si with the desired mesopore structure can also be obtained by several other scalable methods, including chemical etching of metallurgical grade and micron-sized silicon powder that is economically available in large quantities and suitable for large-scale production. The rational design of the novel structure developed in this work may also guide the development of other materials that may experience large volume changes during its operation processes. Sample preparation MSS samples were prepared by electrochemical etching of heavily boron-doped, <100> oriented single crystal Si wafers (<1 mΩ·cm resistivity, Siltronix Inc.) by application of a constant current density of ~225 mA cm −2 for 358 s in an aqueous 48% hydrofluoric acid (HF)/ethanol electrolyte (HF:EtOH=3:1, v-v) [34] . A freestanding film of the MSS was then removed from the crystalline Si substrate by application of a constant current density of ~10 mA cm −2 for 750 s in an aqueous HF/ethanol electrolyte (HF:EtOH=1:30, v-v). The MSS film was washed several times with ethanol, then fractured by ultrasonication in ethanol to form ~40-μm particles, and dried for further use. Carbon coating on the MSS particles was conducted using a vacuum chemical vapour deposition system. The MSS sample was loaded in a tube furnace, which then was evacuated at room temperature to a vacuum level of ≤1 mTorr. The furnace was heated to 600 °C at a rate of 10 °C min −1 , and at 600 °C, the precursor gas (argon: acetylene=9:1) was introduced. The furnace temperature was increased to 690 °C and was maintained at that temperature for 30 min. After carbon deposition, the furnace was cooled to room temperature in pure argon. Structure characterization XRD spectra were obtained on a Philips X’Pert X-ray diffractometer using a Cu K α sealed tube ( λ =1.54178 Å) at 0.5° min −1 . SEM measurement was conducted on an FEI Helios Nanolab dual-beam focused ion beam SEM. After cycling, the samples were obtained from disassembled cells, washed three times with anhydrous dimethyl carbonate, and dried in the antechamber of the glove box under vacuum. Nitrogen sorption isotherms were obtained using a Quantachrome Autosorb automated gas sorption system at −196 °C. Specific surface areas and pore size distributions were calculated using the Brunauer–Emmett–Teller theory and the Barrett–Joyner–Halenda method. Specific pore volumes were measured at a relative pressure of 0.99. In-situ TEM battery experiment In-situ lithiation of the MSS particle was performed using a Nanofactory scanning tunnelling microscopy holder. Assembly of the in-situ TEM nano-cell battery was performed in an argon-filled glove box and transferred to the TEM in an argon-filled glove bag. The turbo pump in the TEM was pre-set to the maximum speed before loading the sample. Once the sample holder was inserted into the TEM, the sample environment was quickly pumped to vacuum. The total air exposure of the sample during loading into the TEM was <2 s. TEM measurements were performed using an FEI Titan operating at an accelerating voltage of 300 kV. During lithiation, a −2 V potential was applied to the working electrode to drive the Li into the Si electrode through the Li 2 O solid electrolyte. Electrochemical measurements The MSS electrode was prepared by mixing an appropriate amount of the carbon-coated MSS sample with Super P (Timcal), and carboxymethyl cellulose sodium salt (Sigma Aldrich) in distilled water to form a slurry, which was then pasted on a copper foil (Pred. Materials International, Inc.). The Si loading in the mixture was kept at 46 and 40 wt%. The binder of carboxymethyl cellulose sodium salt was kept at 20 wt% in all electrodes. After drying in vacuum at 70 °C, the electrodes were tested in coin cells with Li metal as the counter and the reference electrode. The electrolyte was 1 M LiPF 6 in a mixture of ethylene carbonate and dimethyl carbonate in a 1:2 volume ratio with 10 wt% fluorinated ethylene carbonate as electrolyte additive. A microporous membrane (Celgard 3501) was used as the separator. The coin cells were assembled in an argon-filled glove box (MBraun Inc.). All the batteries were tested using galvanostatic charge-discharge protocols on a BT-2000 Arbin Battery Testing System (Arbin Instruments) at room temperature. For the electrodes with low Si loading (~0.5 mg cm −2 ), tests were conducted within a voltage range of 0.05–1.5 V. The batteries were cycled at a current density of 0.1 A g −1 for three cycles and then cycled at 1 A g −1 for long-term cycling stability or at different current densities for rate performance. The current density was calculated on the basis of the MSS weight. All of the specific weight-capacity values in this paper were calculated on the basis of the whole electrode weight including active material, binder and conductive carbon. For the electrodes with high Si loading (~2 mg cm −2 ), tests were conducted within a voltage range of 0.005–1.0 V. The batteries were cycled at a current density of 0.06 mA cm −2 for three cycles and then cycled at 0.75 mA cm −2 for charge (de-lithiation) and 0.5 mA cm −2 for discharge (lithiation). Cyclic voltammograms were measured on a CHI660d workstation (CH instruments, USA). How to cite this article: Li, X. et al . Mesoporous silicon sponge as an anti-pulverization structure for high-performance lithium-ion battery anodes. Nat. Commun. 5:4105 doi: 10.1038/ncomms5105 (2014).